Hybrid nanoparticle–microcavity-based plasmonic nanosensors with improved detection resolution and extended remote-sensing ability Optical nanosensors based on plasmonic nanoparticles have great potential for chemical and biological sensing applications, but their spectral detection resolution is severely constrained by their broad resonance linewidth, and their spatial sensing depth is limited to several tens of nanometres. Here we demonstrate that coupling a strong dipolar plasmonic resonance of a single metallic nanoparticle to the narrow bandwidth resonances of an optical microcavity creates a hybrid mode and discretizes the broad localized resonance, boosting the sensing figure-of-merit by up to 36 times. This cavity–nanoparticle system effectively combines the advantages of Fabry–Perot microresonators with those of plasmonic nanoparticles, providing interesting features such as remote-sensing ability, incident-angle independent resonances, strong polarization dependence, lateral ultra small sensing volume and strongly improved detection resolution. Such a hybrid system can be used not only to locally monitor specific dynamic processes in biosensing, but also to remotely sense important film parameters in thin-film nanometrology. Non-invasive optical characterization of thin film properties such as thickness and optical density, particularly for biomaterials, is usually achieved by using traditional optical microscopy and various spectroscopic techniques such as transmission or reflection spectroscopy [1] or ellipsometry [2] . For all these techniques the minimum lateral sensing areas are determined by the beam diameters used, which are, in a typical experiment, of the order of several micrometres. It is therefore impossible to measure film properties on a lateral nanometre level such as thickness variations, composition inhomogeneities and surface morphology. Single-particle plasmon-resonance-based nanoprobes are ideal tools for spatially sensing nanoscale environment changes such as molecular-binding events [3] , [4] , [5] , catalytic reactions [6] and local electrochemical current [7] , phase-changing processes [8] , [9] and hydrogen gas adsorption [10] , [11] . However, plasmonic nanosensors using localized surface plasmons (LSPs) are inherently insensitive to changes happening outside the evanescent fields of the plasmon resonance itself. The spatial sensing depth into the substrate is therefore restricted to a nanometre thin layer beneath the particle and the material properties of the substrate used can only be determined in that tiny region. Sensors based on propagating surface plasmons fundamentally lack of the ability to determine the location of the sensing event, as the propagating plasmonic mode exchanges energy to a dielectric waveguide mode via intermodal coupling over a characteristic length scale [12] . This means that the information about the spatial position of the sensing event is effectively lost and sensors relying on propagating plasmons are inherently incapable of spatially resolving nanoscale environmental changes. On the other hand, the overall figure-of-merit (FoM) of the sensing response of an LSP-based nanosensor severely suffers from the broad localized plasmonic resonance linewidth because of the large intrinsic absorption of metal in general and the dominant radiative scattering contribution [13] , [14] . To increase the total FoM great efforts have been made to enhance the refractive index sensitivity of individual plasmonic nanoparticles by optimizing their size and shape [15] , [16] , [17] , but very little attention has been drawn to narrow the spectral linewidth. Recently, several new design principles, including plasmon hybridization [18] , transformation optics [19] and subgroup decomposition [20] have been proposed and used to modify the resonance lineshape and enhance the spectral contrast of individual metallic nanodimers and nanoclusters. However, the reduction of the LSP resonance linewidth based on the aforementioned strategies is very limited and the quality factor of hybridized resonances [21] , [22] is still around one order of magnitude smaller than that of propagating plasmons [23] , [24] . Perhaps the largest plasmonic cavity quality factor achieved so far is from a surface-plasmonic whispering-gallery microcavity [25] , which obviously loses the nanoscale detection ability because of its large dimension of several tens of micrometres. Moreover, all these approaches described above usually rely on stringent design and precise control of the arrangement of individual components such as interparticle distance and particle shape, which further impose experimental difficulties (especially in the fabrication) and cannot be applied to many other systems consisting of only one or a few nanoparticles. To overcome these limitations plasmonic nanosensors currently face, we report here the first measurements of an isolated plasmonic nanoparticle–cavity system consisting of a single subwavelength metallic nanoparticle and a micrometer-thick film-type cavity. We reveal the fundamental optical properties of this hybrid system using single-particle dark-field (DF) microscopy and give a detailed theoretical analysis including a straightforward extended Fabry–Perot (FP) model. Finally, we discuss the sensing properties of this structure (related to measuring changes of the optical properties of the substrate on a lateral nanoscale area) and demonstrate them in the experiment by photobleaching the cavity layer using ultraviolet (UV) light. We emphasize that such single-particle measurements are capable of revealing the intermodal coupling process between LSP resonances and FP modes and distinguish their respective contributions to the optical response of the entire hybrid mode. These results are distinctively different from previous studies on cavity-particle ensembles [26] , [27] , [28] , [29] where cavity modes usually dominate the whole spectrum and ultimately result in extremely weak coupling [27] . In particular, we employ the higher-order FP modes, which discretize the broad LSP resonance, and hence strongly enhance the detection resolution of such a hybrid nanoparticle–microcavity probe. Design of an isolated nanoparticle–microcavity system In the optical system investigated here ( Fig. 1a ), the LSP resonance is created by coupling an external electromagnetic (EM) wave to the quasi-free electron ensemble of a subwavelength metallic nanoparticle. The incident light induces the electron ensemble to oscillate with the same frequency as EM wave, and the particle shows a distinct resonance, the so-called LSP resonance (LSPR), at one characteristic frequency. The spectral position of this resonance depends on the shape of the particle, the materials surrounding it and the metal used [13] , [14] . To create a distinct LSPR we used gold nanoparticles with an average diameter of about 100 nm (BBI International) dispersed in water. Gold is an almost ideal metal for creating strong LSPRs as the inherent oscillator damping constant resulting from electron–phonon collisions is one of the lowest of all metals [30] . Preliminary experiments show that these colloidal particles, if deposited on low-loss dielectric substrates, have a dominant dipolar plasmonic resonance in the red part of the visible spectrum (typically at around 600–800 nm) and a much weaker quadrupole resonance more to the blue end of the spectrum. 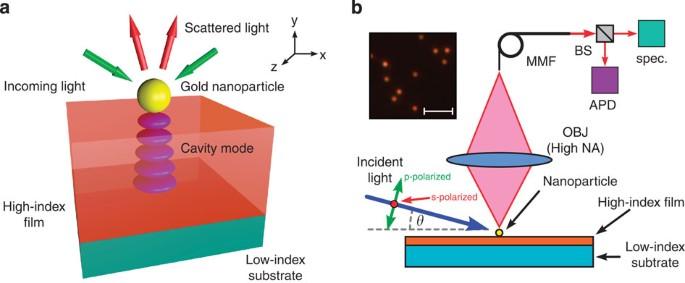Figure 1: The concept of lateral nanosening using a hybrid nanoparticle–cavity system. (a) Single gold nanoparticle on a Fabry–Perot microcavity. The green and red arrows indicate the incident and scattered light, respectively. (b) Confocal dark-field microscope for measuring the scattering spectra of single metallic nanoparticles (MMF, multimode fibre; BS, beam splitter; spec., spectrometer; APD, avalanche photodiode; OBJ, microscope objective). The blue arrow indicates the direction of the incident light (the polarization states are shown by the green and red arrows. The angle of incidence is defined with respect to the film plane (angleθin the figure)). The inset shows a typical dark-field image of the sample. The bright red spots correspond to the gold nanoparticles (scale bar indicates a length of 5μm). Figure 1: The concept of lateral nanosening using a hybrid nanoparticle–cavity system. ( a ) Single gold nanoparticle on a Fabry–Perot microcavity. The green and red arrows indicate the incident and scattered light, respectively. ( b ) Confocal dark-field microscope for measuring the scattering spectra of single metallic nanoparticles (MMF, multimode fibre; BS, beam splitter; spec., spectrometer; APD, avalanche photodiode; OBJ, microscope objective). The blue arrow indicates the direction of the incident light (the polarization states are shown by the green and red arrows. The angle of incidence is defined with respect to the film plane (angle θ in the figure)). The inset shows a typical dark-field image of the sample. The bright red spots correspond to the gold nanoparticles (scale bar indicates a length of 5 μ m). Full size image The microcavities we are using here are basically high refractive index (HI) films with thicknesses of several micrometres located on low-index substrates. Because of the refractive index steps below and above the film, light is reflected at both boundaries and a standing wave pattern, that is, a local cavity mode forms inside the HI film if the circulating beam is able to acquire a phase shift of a multiple of 2 π after two reflections. Such a cavity, which has found applications in many areas of optical science such as wavelength filters [31] or mode selectors [32] , is called a FP cavity. Here, we use two kinds of FP-based microcavities: The first cavity was a 2.64- μ m thick single-crystal bismuth-doped yttrium-iron-garnet (BiYIG) film located on a gadolinium-gallium-garnet (GGG) substrate (thickness 1 mm) (Innovent) and the second one was a 1.27- μ m thick chalcogenide film (Ge 25 Sb 10 Se 65 ) on a borosilicate glass substrate (Schott BK7, thickness 1 mm) [33] , [34] . The optical properties of these films and substrates are described in the Methods section. When an individual metallic nanoparticle is directly deposited on the microcavity surface, cavity and LSPR modes couple to each other at very characteristic frequencies and form hybrid plasmonic supermodes. In such a system the nanoparticle effectively acts as an optical antenna concentrating the EM energy of the incident light into a small volume and redirecting it into the FP cavity modes. During circulating inside the FP cavity, the EM energy is partly transferred out of the cavity modes into the LSPR and is then scattered away from the nanoparticle. Spectroscopic characterization and numerical modelling To investigate the scattering properties of the nanoparticle–cavity system we used DF confocal microscopy ( Fig. 1b ). In such geometry the LSPR is excited by an incident EM wave at a relatively small angle (definition of angle in Fig. 1b ), and the scattered light is collected by an objective above the particle (a true-color DF image of the particle distribution on the BiYIG surface is shown in the inset of Fig. 1b where individual gold nanoparticles are clearly visible; details about the DF spectroscopy are given in the Methods section.). The scattering spectrum of a single gold nanoparticle on the BiYIG sample shows a broad scattering peak with pronounced spectral oscillations modifying it at the long-wavelength edge of the visible spectrum (purple curve in Fig. 2a ). Using the Fourier transformation (FT) analysis described in the Methods, the high-frequency components on the original scattering spectrum (purple curve in Fig. 2a ) have been removed from the FT spectrum and a clear scattering peak at around 750 nm remains (red curve in Fig. 2a ). By simulating the scattering intensity of a comparable particle located on a semi-infinite BiYIG substrate (no lower GGG film), we can identify this main peak as the dipolar LSPR of the gold nanoparticle. The FT analysis can therefore be interpreted as a mathematical operation to remove the lower boundary of the FP film and to reveal the properties of the bare LSPR. This LSPR peak has been approximated by a Lorentzian shape function, giving a linewidth Δλ LSPR of about 140 nm (blue curve in Fig. 2a ), which is approximately seven times larger than the full-width half-maximum spectral width of the fast oscillations Δλ FP (here ≈20 nm). Such a large reduction in the linewidth of each individual resonance implies a significant improvement in the detection resolution limit or an enhanced overall FoM when this hybrid resonance is employed in refractive index sensing applications. Moreover, we observed that the fast oscillations are much more pronounced if the incident light is s-polarized ( Figs 2b,c ). Note that the total spectral linewidth of s-polarized scattering spectrum ( Fig. 2b ) is narrower than that of p-polarized spectrum, which is due to the substrate effect on the nanoparticle scattering response. 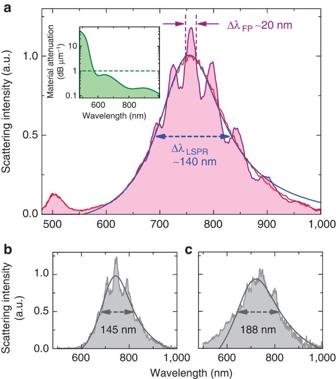Figure 2: Spectral dependence of the scattered light. Measured scattering spectra of one single gold nanoparticle located on the HI-garnet film (film thickness 2.64 μm, particle diameter 100 nm). (a) Dark-field scattering spectrum when unpolarized white-light excitation is used (purple curve). The red curve shows the scattering spectrum after the Fourier analysis and the blue curve represents the corresponding Lorentzian fit. The inset depicts the material absorption of BiYIG. (b) and (c) Measured scattering spectra (grey) and Lorentzian-fit curves (black) when the incident light is polarized ((b) s-polarization, (c) p-polarization). [35] , [36] Figure 2: Spectral dependence of the scattered light. Measured scattering spectra of one single gold nanoparticle located on the HI-garnet film (film thickness 2.64 μm, particle diameter 100 nm). ( a ) Dark-field scattering spectrum when unpolarized white-light excitation is used (purple curve). The red curve shows the scattering spectrum after the Fourier analysis and the blue curve represents the corresponding Lorentzian fit. The inset depicts the material absorption of BiYIG. ( b ) and ( c ) Measured scattering spectra (grey) and Lorentzian-fit curves (black) when the incident light is polarized (( b ) s-polarization, ( c ) p-polarization). Full size image For a qualitative analysis we simulate the scattering properties of a 600-nm thick BiYIG film on GGG with and without gold particle (diameter 100 nm), and compare the relative scattering intensities induced by the FP-cavity Δ I ( Fig. 3a ), which in fact gives directly the enhancement/suppression factor relative to the case when no cavity is present. Without particle, Δ I = (I FP / I SL )−1 (scattering intensities of cavity and of single BiYIG layer: I FP and I SL ) and for the nanoparticle–cavity system Δ I = (I FP−LSPR / I LSPR )−1 (scattering intensity of particle–cavity system and of a similar gold particle on a semi-infinite BiYIG substrate: I FP−LSPR and I LSPR ). The spectral distributions of Δ I of cavity and particle–cavity systems are significantly different ( Fig. 3a ), revealing that the gold nanoparticle has a distinct influence on the cavity's optical response. The light intensity distribution inside the cavity at one of the resonances is depicted in Fig. 3b (616 nm, dashed red line in Fig. 3a ), showing that the EM field below the particle is strongly enhanced and a FP-type mode is excited inside the HI layer. The spatial extension of that cavity mode along the x direction is of the order of the particle diameter (≈100 nm). There is no indication of a significant EM field outside this area, meaning that the cavity mode is localized below the nanoparticle inside a nanoscale cylinder having its axis along the y direction. It has to be mentioned that a strong coupling between particle and FP cavity is observed only if the refractive index of cavity layer is > 2 (that is, the index of semi-infinite substrate). 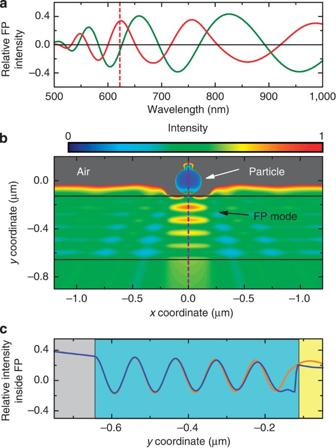Figure 3: Electromagnetic simulation of the nanoparticle–cavity system. (a) Comparison of the spectral distributions of the relative FP amplitude of the scattered light by the particle–cavity system (red) and the same cavity without particle (green). The calculations have been performed using finite-difference-time-domain simulations. (b) Intensity distribution of a cross section of the particle–cavity system at an excitation wavelength of 616 nm (corresponds to the vertical dotted red line ina). The intensity ranges from low (blue) to high (red). To reveal the features of the cavity mode, the intensity in the air region has been set to a constant value (grey). The black solid lines are guide-to-the-eye to show the boundaries of the HI layer and the coordinates are defined in Fig. 1a. (c) Comparison of the relative intensity distributions (relative to the case without the lower boundary of the FP cavity) of the particle–cavity system (blue) and the bare FP cavity (orange) along the vertical dashed purple line ofb. The coloured backgrounds indicate the different materials (yellow: gold, cyan: BiYIG, grey: GGG). Figure 3: Electromagnetic simulation of the nanoparticle–cavity system. ( a ) Comparison of the spectral distributions of the relative FP amplitude of the scattered light by the particle–cavity system (red) and the same cavity without particle (green). The calculations have been performed using finite-difference-time-domain simulations. ( b ) Intensity distribution of a cross section of the particle–cavity system at an excitation wavelength of 616 nm (corresponds to the vertical dotted red line in a ). The intensity ranges from low (blue) to high (red). To reveal the features of the cavity mode, the intensity in the air region has been set to a constant value (grey). The black solid lines are guide-to-the-eye to show the boundaries of the HI layer and the coordinates are defined in Fig. 1a. ( c ) Comparison of the relative intensity distributions (relative to the case without the lower boundary of the FP cavity) of the particle–cavity system (blue) and the bare FP cavity (orange) along the vertical dashed purple line of b . The coloured backgrounds indicate the different materials (yellow: gold, cyan: BiYIG, grey: GGG). Full size image The circulating cavity mode undergoes a complex reflection process below the nanoparticle, as the relative intensity distribution shows a step-function-like behaviour across the metal-dielectric boundary (blue curve in the cross section plot in Fig. 3c ), which is completely different from the bare cavity (orange curve in Fig. 3c ). The relative intensities here are defined in a similar way as described above, but are plotted as a function of the y coordinate at a fixed wavelength of 616 nm (coordinate system defined in Fig. 1a ). This proves that we excite hybrid plasmonic modes consisting of a dipolar LSPR coupled to the individual modes of the microcavity. In other words, we are able to couple a nanoscale Lorentzian-type plasmonic oscillator to purely optical cavity modes, leading to a discretization of the LSPR scattering spectrum. It has to be pointed out that this coupling process can either enhance or suppress the scattering intensity of the nanoparticle by up to ±40% ( Fig. 3a ). The stronger oscillations for s-polarized input light result from the fact that the circulating beam inside the FP cavity requires a transverse electric field distribution, which in fact are much smaller for p-polarized incident light. The oscillations in the LSPR spectrum are less pronounced at shorter wavelengths, coming from the increasing material absorption of BiYIG towards shorter wavelengths. For λ 0 <600 nm, the loss of BiYIG exceeds 1 dB μ m −1 (inset of Fig. 2a ) and a cavity mode cannot be formed as a significant fraction of the EM energy of the circulating beam is absorbed before it reaches its first reflection at the BiYIG/GGG junction. Description by an extended FP model To theoretically describe the spectral response of the particle–cavity system, we apply an extended FP-resonance model, which takes account of the specific properties of light reflection below the metal particle [37] . This model has been used for analysing the reflection properties of specific optical devices such as photonic crystal mirrors or cavities [38] . It basically assumes that the metallic particle induces an additional phase shift φ M to the reflected beam and elongates the penetration depth of the EM wave into the upper interface by a distance Δ d ( Fig. 4a ). 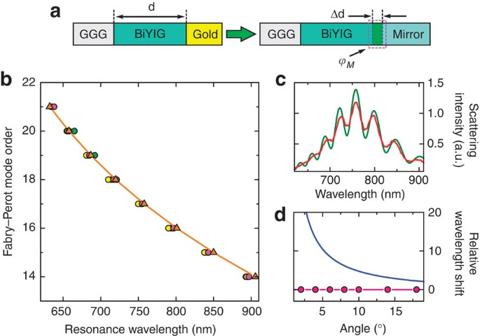Figure 4: The extended Fabry–Perot model. (a) Schematic of the extended FP structure. The original gold layer (left-handed image) has been assumed to extend the cavity by Δd and induces an additional phase shiftφM(highlighted by the dashed purple box in the right-handed image). (b) Experimentally measured FP resonances (peaks in the scattering spectra) as a function of mode order. The circles correspond to four different nanoparticles on the BiYIG film, each colour referring to one single particle. The four particles were randomly selected for measurements, demonstrating the highly reproducible spectral-response of our particle–cavity system. The orange triangles show the calculated resonance positions obtained from our FP analysis (the orange line is a guide-to-the-eye). (c) Example scattering spectrum of one of these nanoparticles (unpolarized excitation, red line) and the corresponding calculated scattering intensity using the FP approach (green line). (d) Relative resonance shift of the 750 nm resonance if the angle of the incident light is changed (angle defined with respect to the plane of the FP film, ΔλR=(λR(θ)−λR(0°))/λR(0°)). The pink dots correspond to the measured resonance values of the nanoparticle–cavity system, the blue curve to a bare Fabry–Perot without particle. In this model, the resonance condition for having a maximum in reflection is given by: Figure 4: The extended Fabry–Perot model. ( a ) Schematic of the extended FP structure. The original gold layer (left-handed image) has been assumed to extend the cavity by Δd and induces an additional phase shift φ M (highlighted by the dashed purple box in the right-handed image). ( b ) Experimentally measured FP resonances (peaks in the scattering spectra) as a function of mode order. The circles correspond to four different nanoparticles on the BiYIG film, each colour referring to one single particle. The four particles were randomly selected for measurements, demonstrating the highly reproducible spectral-response of our particle–cavity system. The orange triangles show the calculated resonance positions obtained from our FP analysis (the orange line is a guide-to-the-eye). ( c ) Example scattering spectrum of one of these nanoparticles (unpolarized excitation, red line) and the corresponding calculated scattering intensity using the FP approach (green line). ( d ) Relative resonance shift of the 750 nm resonance if the angle of the incident light is changed (angle defined with respect to the plane of the FP film, Δλ R =( λ R ( θ )− λ R (0°))/λ R (0°)). The pink dots correspond to the measured resonance values of the nanoparticle–cavity system, the blue curve to a bare Fabry–Perot without particle. Full size image with the FP-mode order number m , the resonance wavelength λ R , and the refractive index and thickness of the HI layer n HI and d , respectively. Both phase shift and cavity elongation have been determined for the simulated example discussed here (referring to the structure investigated in Fig. 3 ) by matching the resonance wavelengths from equation (1) to all visible FP resonances of the simulated system (maxima of the red curve in Fig. 3a ). This matching procedure additionally requires finding the correct mode order numbers for each resonance, which has been done by successively increasing m in equation (1) and coarsely matching the resonances. In a next step, the optimal combination of the two free parameters in equation (1) (phase shift and cavity elongation) has been determined by looking for that combination of φ M and Δd giving the smallest standard deviation (s.d.) σ λ (see Supplementary Methods for details, s.d. defined by Supplementary equation S1 ). The analysis shows the optimal parameter combination is given by φ M =0.39×2 π and Δ d =41.6 nm with σ λ =0.95 nm. This small s.d. reveals that our model describes the spectral positions of the resonances of the cavity–nanoparticles system within accuracy better than ±1 nm. Figure 4b compares the measured spectral positions of the scattering peaks of four different nanoparticles on the BiYIG sample. Clearly, all particles show the FP resonances at the same spectral positions, making our system independent of the actual shape of the LSPR used. Using the experimentally measured thickness of the BiYIG film, the extended FP model equation (1) has been utilized to calculate the resonances. The calculations match the experimentally measured resonances extremely accurately ( Fig. 4b ). This is a remarkable result, as both the φ M and Δ d have been determined from the qualitative finite-difference-time-domain simulations in which a much smaller HI-film thickness was considered, and not from the experiment. It has to be pointed out that if phase shift and cavity elongation are virtually set to zero, all resonances shift far off the measured ones (by about 15 nm to shorter wavelengths), which clearly shows that the HI cavity is strongly influenced by the presence of the nanoparticle. The physical details of the reflection process are rather sophisticated, as the particle forms a non-planar mirror on the BiYIG film. However, all these effects are automatically included into the extended FP model. It has to be pointed out that if the cavity elongation is ignored, that is, Δ d =0 nm (as for example, equation (1) in ref. 30 ), the above described fitting procedure gives σ λ =9.39 nm ( φ M =0.62×2π), which is 10 times less accurate than if Δ d is included. Therefore, the inclusion of the cavity elongation parameter is key to reveal the physics behind the coupling mechanism of plasmonic and cavity modes in the film–nanoparticle system. Using the reflectivities of a FP-cavity R FP and a single BiYIG layer R 1 (both equations can be found in ref. 1 ), the scattering intensity of our investigated particle–cavity system has been calculated by the following equation: with the vacuum wavelength λ 0 . The calculated scattering spectrum agrees very well with the experimental one ( Fig. 4c ) and thus equation (2) can be used to simulate the scattering properties of a nanoparticle–cavity system in a straightforward way without using any sophisticated calculation technique. It has to be pointed out that equations (1) and (2) describe the behaviour of such a cavity–nanoparticle system qualitatively and quantitatively for both spectral position of the resonances and scattering intensity analytically, which in fact makes both equations extremely useful for any real-world applications. In a future publication we are planning to simulate other cavity–nanoparticle systems having various particle shapes (two examples shown in the Supplementary Table S1 ) and apply equations (1) and (2), as our model is a very useful and straightforward-to-use tool to systematically investigate such nanoscale hybrid optical system. Angle-resolved measurements reveal that the spectral positions of the hybridized resonances are independent of the incidence angle (0°< θ <20°, incidence angle defined Fig. 1b ). This independence is very different compared with a bare FP without particle (relative changes of one of the resonances are shown in Fig. 4d ). For the angles investigated here the bare FP resonances would shift by a factor of 20, whereas the resonances of the nanoparticle–cavity system remain at the same spectral positions. This again shows that LSPR and cavity mode are interacting via intermodal coupling and form a hybrid plasmonic supermode. Sensing the photobleaching dynamics using the nanosensor The fast oscillations in the scattering spectrum ( Fig. 2a ) are spectrally much narrower than the LSPR (about seven times), which allows using our nanoparticle–microcavity system for ultra-precisely sensing the optical properties of the HI layer on a very small lateral area. The spectral positions of the fast oscillations are effectively independent of the material on top of the HI layer, and the sensing performance of our system is thus maintained even in an environment which changes with time. It is actually possible to sense simultaneously changes of the upper material using the LSPR and of the film using the sharp FP resonances, both on a lateral nanoscale area. A comparison of the sensitivities (slope of the scattering intensity with respect to wavelength) of nanoparticle-cavity and bare LSPR ( Fig. 5a ) shows that the slope of our system can be 3.6 times steeper than that of the bare LSPR, leading to a significantly improved sensing capability. Using equation (1) and the experimentally measured spectral width of the fast oscillations Δ λ FP (shown in the inset of Fig. 5b ), we define a FoM parameter (on the basis of the definition given in ref. 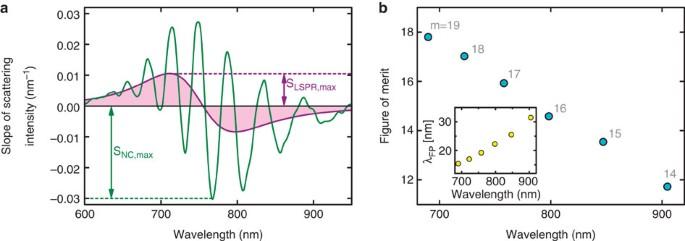Figure 5: Sensing properties of the nanoparticle–microcavity system. (a) Distribution of the spectral derivative of the scattering intensity as a function of wavelength of the investigated Au-BiYIG nanoparticle–cavity system (green curve). The purple curve shows the derivative of the corresponding Lorentzian-fit function of the localized surface plasmon resonance. (b) FoM sensing value as function of wavelength (measured). The grey numbers refer to the FP-mode order number m. The lower left-handed inset shows the spectral width of the FP resonances as a function of wavelength. 39 ) for sensing changes of the real part of the refractive index of the HI layer (lateral nanoscale volume sensing FoM): Figure 5: Sensing properties of the nanoparticle–microcavity system. ( a ) Distribution of the spectral derivative of the scattering intensity as a function of wavelength of the investigated Au-BiYIG nanoparticle–cavity system (green curve). The purple curve shows the derivative of the corresponding Lorentzian-fit function of the localized surface plasmon resonance. ( b ) FoM sensing value as function of wavelength (measured). The grey numbers refer to the FP-mode order number m. The lower left-handed inset shows the spectral width of the FP resonances as a function of wavelength. Full size image Across the entire LSPR (>140 nm), our system shows FoM values >12 ( Fig. 5b ), which in fact represents a significant improvement compared with other individual finite nanostructures, which hardly reach FoM > 6 (refs 22 , 41 ). The maximum FoM we can reach with our nanoparticle–cavity system is 18 compared with just 0.5 in the case of a semi-infinite substrate, that is, when there is no cavity present. The simulations show that the maximum FoM, which is obviously reached when the particle is homogenously embedded in BiYIG is 4.5. Therefore, our coupled system uniquely allows boosting the sensing performance of localized plasmonic systems by a factor of 36 if the optical properties of the layer below the particle are to be measured. The FoM increases towards shorter wavelength—a result of the reduced spectral width of the resonances, which effectively overcompensates the contribution of the increasing FP-mode order number. Even higher FoM values can be achieved by using thicker HI films. Then the light travelling inside the cavity needs more time to accomplish one complete round trip and thus accumulates more phase during propagation, hence being more sensitive to changes of the refractive index. However, the overall limiting factor of the FoM will be the material attenuation of the HI layer, as at least one complete round trip is required to form a standing wave pattern, that is, a cavity mode. It is important to note that many oscillations, that is, higher-order FP resonances are observed across the LSPR. Analysing the sensing properties of each of these resonances can reveal the complex dielectric function (refractive index dispersion and absorption) of the substrate material in a lateral nanoscale area. A more detailed analysis and a route to optimize the performance of FP–LSPR systems will be given in future publications. As a sensing example, we investigate the influence of UV photobleaching on the FP resonances of gold nanoparticles on a chalcogenide film (scattering intensity of the nanoparticle-chalcogenide sample is shown in Fig. 6b ). We observe a linear shift of the resonances to shorter wavelength for increasing UV doses ( Fig. 6a ), with a maximum shift of about 4 nm (the spectra of unbleached and fully bleached sample in proximity of the 700 nm resonance are shown in inset of Fig. 6 ), which is consistent with the shift observed in the bulk film ( Supplementary Fig. S1 ). Assuming that the smallest measureable spectral wavelength shift, which can be resolved from the scattering measurements ( Fig. 6 ) is Δλ =0.5 nm, the smallest detectable refractive index change of the substrate is calculated to be 1.75×10 −3 (Profilometer measurements, with a step height repeatability of 6Å and a noise floor below 1nm RMS as measured on the scan stage, show that the thickness of bleached and unbleached film are identical). The observed blue shift could be explained by two facts: first the film undergoes a significant densification during UV exposure, which ultimately leads to a reduction of the film thickness. Moreover, as the photobleaching is performed under air, oxyselenide molecules can form inside the film and defects inside the glass matrix, like homopolar bond type, can be mitigated. The last phenomenum leads to a blue shift of the electronic band-gap of the chalcogenide which, consequently, reduces the film's refractive index [40] . According to equation (1), both effects give rise to a shift of the FP resonances to shorter wavelengths. The spectra of the scattering intensity of the bare bleached and unbleached FP film (without particle) show, as expected, no FP-related oscillations ( Fig. 6c ). Obviously, the nanoparticle is required to couple the light into the FP layer, clearly showing the importance of the hybrid particle–cavity system for lateral nanoscale volume sensing. 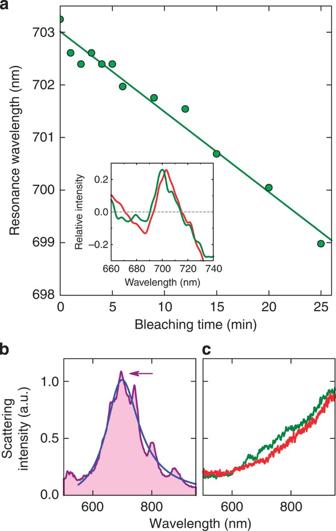Figure 6: Proving the concept of nanoscale sensing by ultraviolet photobleaching. (a) Spectral shift of one of the FP resonances of the gold nanoparticle–chalcogenide system as a function of photobleaching time (particle diameter: 100 nm, film thickness: 1.27μm, nominal chalcogenide composition: Ge25Sb10Se65). The green line is a linear fit to the data points. The inset shows the relative FP intensity (normalized by the corresponding Lorentzian LSPR function) in the vicinity of the 700 nm resonance before (red) and after (green) bleaching. (b) Example scattering spectrum (purple) together with the Lorentzian approximation (blue). The purple arrow indicates the investigated FP resonance. (c) Measured scattering intensity of the chalcogenide surface without particle (green: bleached, red: unbleached). Figure 6: Proving the concept of nanoscale sensing by ultraviolet photobleaching. ( a ) Spectral shift of one of the FP resonances of the gold nanoparticle–chalcogenide system as a function of photobleaching time (particle diameter: 100 nm, film thickness: 1.27 μ m, nominal chalcogenide composition: Ge 25 Sb 10 Se 65 ). The green line is a linear fit to the data points. The inset shows the relative FP intensity (normalized by the corresponding Lorentzian LSPR function) in the vicinity of the 700 nm resonance before (red) and after (green) bleaching. ( b ) Example scattering spectrum (purple) together with the Lorentzian approximation (blue). The purple arrow indicates the investigated FP resonance. ( c ) Measured scattering intensity of the chalcogenide surface without particle (green: bleached, red: unbleached). Full size image In conclusion we have reported on a new kind of plasmonic system consisting of a subwavelength metallic nanoparticle located on a FP-type microcavity. This structure reveals a special type of optical mode with strong oscillations (up to 40%) in the scattering peak spectrum of the LSPR. These oscillations are associated with intermodal coupling between LSPR and cavity modes, leading to a new type of hybrid plasmonic resonance. The resonances are independent of the incident angle and are excited dominantly in one polarization direction. Time-domain simulations show that these hybrid modes have a distinct EM-field enhancement below the particle with a lateral extension of about 100×100 nm 2 . All relevant optical properties of the nanoparticle–cavity system have been described on the basis of a straightforward extended FP model, taking into account the sophisticated reflection process at the particle-layer boundary. We observe a strong sensitivity enhancement and show one sensing example based on UV photobleaching of a chalcogenide film. We expect our device to find applications in several areas: because of the strong lateral field confinement, our system is able to sense the optical properties of thin films on very small scale, which can be useful for detecting local composition variation or thickness irregularities. As the resonances are independent on incident angle, our system can improve current schemes for light harvesting in photovoltaics and in energy recycling. Also applications for modulating localized plasmonic resonances (with for example, piezo- or electro-optics) or in nanoscale lasing can be anticipated. As a next step, we plan to use much smaller nanoparticles with diameters of a few tens of nanometres. Such small particles will allow ultrasmall plasmonic sensing on a lateral nanoscale of just 10 nm 2 or even less, which is far beyond what is possible with currently used plasmonic sensing schemes. Moreover, we are aiming for investigating single flat nanodiscs on HI–FP cavities, which is expected to show a stronger coupling between LSPR and FP modes because of the larger interaction area, thereby enhancing the sensing performance even further. Higher-order LSPRs, higher-finesse cavities and even dielectric multilayers with predefined reflection and transmission characteristics will be considered in future studies to tune the device performance and to engineer the scattering response of nanoparticles in a desired manner, for example, for nanoscale narrow bandwidth plasmonic band-pass or notch filters. A further prospect of the presented scheme is to use active FP films for externally modulating the scattering intensity or to employ materials with large gain for planar single-mode nanolasers. Nanoparticle–microcavity fabrication Gold nanoparticles were deposited on the HI films by a drop-casting process: first the substrate was heated up to 150 °C on a hot-plate. Then a single droplet of the colloidal solution was drop casted onto the hot film and the sample was removed from the hot plate after 2 min of heating. The comparably high temperature (>100 °C on the film surface) leads to a fast evaporation of the water avoiding particle clustering. The nanoparticle concentration of the solution has been adjusted such that the deposited particles are sufficiently spaced apart preventing optical interaction between two neighbouring particles. Optical properties of HI films and substrates The refractive index of BiYIG film and GGG substrate range from 2.86 to 2.37 and from 1.99 to 1.95, respectively, in the spectral interval from 450 to 1,000 nm (refs 41 , 42 ). The BiYIG shows a significant material absorption up to 600 nm of more than 1 dB μ m −1 (inset of Fig. 2a ), whereas the GGG is transparent throughout the entire visible spectrum. The second investigated FP cavity was a 1.27- μ m thick chalcogenide film (Ge 25 Sb 10 Se 65 ) on a borosilicate glass substrate. The refractive index of the chalcogenide film varies from 2.8 to 2.6 for 650 nm < λ 0 < 1,000 nm (ref. 34 ), whereas the index of the BK7 glass substrate changes only slightly from 1.53 to 1.51 (ref. 43 ). The film strongly absorbs for λ 0 < 600 nm as there the electronic bandgap of the chalcogenide starts to play a significant role. Single-particle DF scattering measurements For the DF spectroscopy we mount our samples to a high-precision multi-axis stage (resolution: 10 nm) for lateral sample scanning. The probe light, either emitted by the internal microscope light bulb or an external light source, is gently focused onto the HI film and the scattered light is collected by high-NA objective [36] . This collected light is then coupled into the core of the multimode fibre, which effectively acts as a pinhole for the confocal scan. At the output of the multimode fibre the light is split between an Avalanche Photodiode and a high-sensitivity spectrometer. This arrangement allows selecting one desired nanoparticle on the sample surface and measuring its optical properties individually. Polarization sensitive measurements have been carried out by placing a high-contrast polarizer just before the sample, allowing precise excitation with either p- or s-polarized light. The angle-dependence of the particle's scattering properties have been determined by changing the input angle between 0° and 18° with an accuracy better than 0.5°. The scattering intensity I S has been calculated by subtracting the dark counts from the corresponding raw scattering spectrum and dividing the result by a reference. To decompose the resulting spectra into their individual features, the spectra have been subjected to a detailed FT analysis. The individual contributions to the overall scattering spectrum have been revealed by setting the amplitudes of specific frequency intervals in the FT data to zero, and performing a subsequent inverse FT. Finite-difference-time-domain simulations We use a commercially available FDTD solver (Lumerical Solutions) to simulate the scattering intensity of various substrate geometries including the exact dielectric functions of all materials involved (BiYIG [41] , GGG [42] , gold [44] ). Considering the extremely large difference in the structure dimensions (a micrometer-scale cavity and a 100-nm nanoparticle), two-dimensional simulations for a nanowire of 100 nm diameter on top of 600 nm BiYIG on a semi-infinite GGG substrate were performed to have a qualitative explanation of the observed features. A total-field-scattering-field source was used to illuminate the nanoparticle–cavity system at normal incidence and allows isolating the scattered fields by the particle from the directly reflected fields by the substrate. Electric field intensity distributions were recorded within the illumination area at respective wavelengths by a two-dimensional field profile monitor. Other systems such as the bare BiYIG cavity, Au nanoparticle on semi-infinite BiYIG and a bare semi-infinite GGG substrate were simulated in the same way. How to cite this article: Schmidt, M.A. et al . Hybrid nanoparticle-microcavity based plasmonic nanosensors with improved detection resolution and extended remote-sensing ability. Nat. Commun. 3:1108 doi: 10.1038/ncomms2109 (2012).